Energetics of activation of GTP hydrolysis on the ribosome Several of the steps in protein synthesis on the ribosome utilize hydrolysis of guanosine triphosphate (GTP) as the driving force. This reaction is catalyzed by translation factors that become activated upon binding to the ribosome. The recently determined crystal structure of an elongation factor-Tu ternary complex bound to the ribosome allows the energetics of GTP activation to be explored by computer simulations. A central problem regards the role of the universally conserved histidine, which has been proposed to act as a general base for guanosine triphosphate hydrolysis. Here we report a detailed energetic and structural analysis of different possible protonation states that could be involved in activation of the reaction. We show that the histidine cannot act as a general base, but must be protonated and in its active conformation to promote GTP hydrolysis. We further show that the sarcin-ricin loop of the ribosome spontaneously drives the histidine into the correct conformation for GTP activation. Protein synthesis on the ribosome involves a number of different subprocesses, namely initiation of translation, protein elongation, termination and ribosome recycling [1] , [2] . All of these are dependent on guanosine triphosphate (GTP) hydrolysis by auxiliary protein factors known as translational GTPases. For example, during the bacterial peptide chain elongation cycle where new messenger RNA (mRNA) codons are successively translated, elongation factor Tu (EF-Tu) delivers aminoacyl-transfer RNA (tRNA) to the ribosome in a ternary complex with GTP. Correct matching between the mRNA codon and the tRNA anticodon then leads to the rapid hydrolysis of GTP on EF-Tu, release of EF-Tu·GDP (guanosine diphosphate) and eventually to peptide bond formation with the newly delivered amino acid. Likewise, unidirectional translocation of the ribosome along the mRNA requires the binding of elongation factor G (EF-G) in complex with GTP and subsequent hydrolysis of the GTP molecule. The translational GTPases are generally poor catalysts of hydrolysis by themselves, but become activated for rapid catalysis in complex with the ribosome. The process by which the GTPases are activated has been enigmatic, although components such as the universally conserved ribosomal sarcin-ricin loop (SRL) and invariant His84 ( Escherichia coli EF-Tu numbering) of the translational GTPases have been identified as being important for GTPase activation [3] , [4] , [5] , [6] , [7] . A major breakthrough for understanding the activation process was recently achieved by the determination of the crystal structure of EF-Tu in ternary complex bound to the 70S Thermus thermophilus ribosome [8] . This structure, has the non-hydrolyzable analogue GDPCP (β,γ-methyleneguanosine 5′-triphosphate) replacing GTP in the active site. It suggests that A2662 of the SRL reorients His84 compared with its position in free EF-Tu, such that the histidine coordinates a water molecule for in-line attack on the γ-phosphate of GTP ( Fig. 1a ). This led to the proposal that His84 acts as a general base for activating the water nucleophile in GTP hydrolysis on the ribosome [8] . It was, however, recently argued that such a mechanism is unlikely for a number of reasons [9] . (i) The presence of several negative charges in the immediate vicinity of His84 means that its p K a is likely to be elevated, so that its sidechain is protonated (positively charged) in the reactant state captured in the crystal structure. (ii) The short distance between the nucleophilic water molecule and one of the oxygens of the γ-phosphate strongly suggests that there exists a hydrogen bond between the water and phosphate ( Fig. 1a ). This implies that the water molecule is oriented with its hydrogen atoms pointing away from His84, as a second H-bond with the carbonyl oxygen of Thr61 is also evident. Hence, the close contact between the water and N δ1 of His84 indicates that the histidine donates an H-bond to the water molecule and is thus doubly protonated, as its other sidechain nitrogen donates an H-bond to the phosphate group of A2662. (iii) The hydrolysis reaction with the analogue GTP-γ-S shows no pH dependence over the 6.5–8.5 pH range [5] , in contrast to what would be expected with a general base ionizing in this pH range. (iv) While the mutation of His84 to alanine essentially abolishes GTP hydrolysis, the corresponding mutation to glutamine only moderately reduces the rate of GTP hydrolysis [6] , [7] . This is consistent with the requirement for H-bond donation to the attacking water but inconsistent with the need for a general base, as that function cannot be fulfilled by glutamine. (v) Finally, hydroxide ion attack (generated by proton transfer to His84) on the doubly negatively charged γ-phosphate is expected to be very slow due to strong electrostatic repulsion (in line with the postulated resistance of phosphate dianions to hydroxide attack at the phosphorus center [10] ). 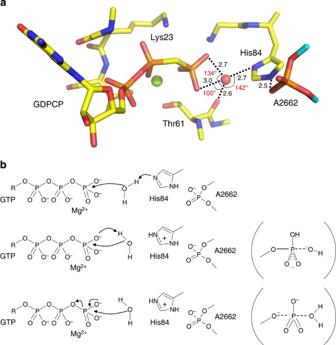Figure 1: The GTPase active site in EF-Tu and possible hydrolysis mechanisms. (a) The crystallographic structure with EF-Tu and the non-hydrolyzable GTP analogue GDPCP bound to the ribosome8is shown with the geometry around the catalytic water molecule (red sphere) indicated. The Mg2+ion bound between the β- and γ-phosphate groups is shown as a green sphere. (b) Three possible hydrolysis mechanisms corresponding to His84 acting as a general base, a stepwise substrate-assisted mechanism and a dissociative path involving expulsion of metaphosphate, both of the latter with His84 protonated. The different nature of the transition states in the associative and dissociative cases with His84 protonated are indicated by the structures within parentheses. Figure 1: The GTPase active site in EF-Tu and possible hydrolysis mechanisms. ( a ) The crystallographic structure with EF-Tu and the non-hydrolyzable GTP analogue GDPCP bound to the ribosome [8] is shown with the geometry around the catalytic water molecule (red sphere) indicated. The Mg 2+ ion bound between the β- and γ-phosphate groups is shown as a green sphere. ( b ) Three possible hydrolysis mechanisms corresponding to His84 acting as a general base, a stepwise substrate-assisted mechanism and a dissociative path involving expulsion of metaphosphate, both of the latter with His84 protonated. The different nature of the transition states in the associative and dissociative cases with His84 protonated are indicated by the structures within parentheses. Full size image It has further been suggested by Voorhees et al . [11] that elevation of the p K a of His84 would not occur until the sidechain of this residue has been repositioned into the GTPase centre. Accordingly, it would become an even better base for abstracting a proton to activate the nucleophile. While such an argument may initially sound attractive, it implies a problematic time-sequence of events. That is, while histidine protonation is very rapid once the ionized form becomes stabilized by the ribosome environment, the proposal assumes that the water molecule protonating His84 will remain in the GTPase centre and that the resulting hydroxide ion can be ‘trapped’ near the γ-phosphate long enough for the relatively slower nucleophilic attack to occur. However, as binding of a hydroxide ion close to a doubly negatively charged phosphate is likely to be very unstable, it is difficult to imagine that this hydroxide ion would not be exchanged for a solvent water molecule on a faster timescale than that of the hydrolysis reaction. In terms of the crystal structure [8] , the general base mechanism would mean that either His84 is still deprotonated in this structure (in which case its p K a is not elevated), or that a hydroxide ion is trapped in the crystal structure near the γ-phosphate, with a protonated histidine (that is, however, essentially neutralized by the phosphate of A2662). In light of the arguments above, it seems more reasonable that the resting (reactant) state of the ribosome complex corresponds to a water molecule residing between the γ-phosphate and a protonated histidine [9] . This scenario suggests that attack of water on the phosphate eventually involves proton transfer from the water molecule to one of the phosphate oxygens rather than to the histidine. The two limiting cases of such a mechanism, corresponding to associative and dissociative pathways are depicted in Fig. 1b , where the former involves proton transfer to a non-bridging phosphate oxygen followed by hydroxide ion attack in a stepwise manner [12] , [13] . The limiting case for a dissociative mechanism, on the other hand, corresponds to expulsion of metaphosphate followed by neutral water attack ( Fig. 1b ). Eventually proton transfer to the GDP leaving group would take place either through a non-bridging oxygen or additional water molecules [12] , [13] . An associative substrate-assisted mechanism has been proposed for other GTPases [14] , [15] , [16] and was recently explored by Adamczyk and Warshel [17] for EF-Tu, who concluded that the effect of His84 is mainly allosteric. However, in order to distinguish between the different mechanistic alternatives above and, in particular, to address the question whether His84 acts as a general base, it is paramount to evaluate the energetics of the possible protonation states involved. In this work, we have used extensive molecular dynamics (MD) computer simulations, utilizing the free energy perturbation (FEP) technique [18] , to compare the energetics of the following possible processes in the GTPase centre of the ribosome, relative to their energetics in aqueous solution: Here, His 0 and HisH + denote the neutral and protonated forms of His84, respectively, and represents the GTP molecule. Process (1) thus corresponds to His84 acting as a general base as proposed by Voorhees et al . [8] , while (2) and (3) denote proton transfer to the phosphate group in a substrate-assisted mechanism [9] , [17] in presence of either the ionized or the neutral forms of His84, respectively. The last process (4) does not involve any proton transfer but represents expulsion of metaphosphate from GTP as the limiting case of a fully dissociative path. We show that the histidine does not act as a general base, but is protonated in its active conformation to promote GTP hydrolysis. We also show that the SRL of the ribosome spontaneously drives the histidine into the correct conformation for GTPase activation. Structural comparisons The starting point for all simulations in this work was the 3.2 Å resolution crystallographic structure of the ribosome bound EF-Tu ternary complex obtained by Vorhees et al . [8] (see Methods ). As this structure contains neither ions nor water molecules (with the exception of the catalytic water and GTP bound Mg 2+ ion), interior solvent molecule positions were taken as far as possible from two structures of free EF-Tu ternary complexes (PDB codes: 2C78, 1EXM) [19] , [20] . These independent high-resolution (1.4 Å) protein structures are essentially identical, and show a remarkable coincidence of water molecule positions ( Fig. 2a ). Interestingly, the GTP binding region, including the loop containing His84, also superimpose very well onto the ribosome bound structure ( Fig. 2b ), indicating that no large active site rearrangements are required for catalysis [8] . The notable exception is the sidechain of His84, which is in the inactive conformation in the two structures of free EF-Tu ternary complexes. As can be seen from Fig. 2b there are also some differences in the backbone peptide plane orientations immediately around His84, but these differences do not appear to be strongly supported by the 3.2 Å resolution electron density calculated here from the experimental structure factors (see below). 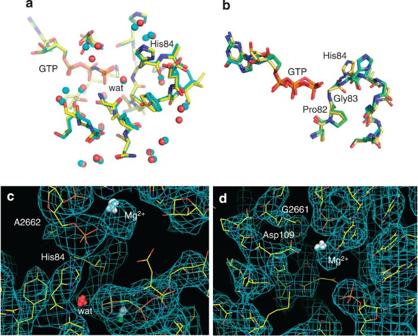Figure 2: Structural comparisons of the GTPase centre. (a) Two independent high resolution crystallographic structures of the free EF-Tu ternary complex19,20(carbon atoms in yellow19and cyan20and waters in red19and cyan20, respectively) show a high degree of coincidence of solvent molecule positions. The position of the catalytic water (‘wat’) is virtually identical to that in the ribosome complex8(where it is the only modelled solvent molecule). (b) Superposition of crystal structures of the ribosome bound8(yellow carbons) and free19,20EF-Tu ternary complexes (cyan and green carbons), illustrating the conformational change of His84 upon activation. (c,d) Comparison of predicted Mg2+ion positions near the GTPase centre from multiple MD simulations (white spheres) with the experimental electron density map. Ion positions can be seen to coincide well with electron density peaks (c) between the phosphates of A2662 and G2663 and (d) between the phosphate of G2661 and Asp109 of EF-Tu. The crystallographic model is shown with solid lines. Figure 2: Structural comparisons of the GTPase centre. ( a ) Two independent high resolution crystallographic structures of the free EF-Tu ternary complex [19] , [20] (carbon atoms in yellow [19] and cyan [20] and waters in red [19] and cyan [20] , respectively) show a high degree of coincidence of solvent molecule positions. The position of the catalytic water (‘wat’) is virtually identical to that in the ribosome complex [8] (where it is the only modelled solvent molecule). ( b ) Superposition of crystal structures of the ribosome bound [8] (yellow carbons) and free [19] , [20] EF-Tu ternary complexes (cyan and green carbons), illustrating the conformational change of His84 upon activation. ( c , d ) Comparison of predicted Mg 2+ ion positions near the GTPase centre from multiple MD simulations (white spheres) with the experimental electron density map. Ion positions can be seen to coincide well with electron density peaks ( c ) between the phosphates of A2662 and G2663 and ( d ) between the phosphate of G2661 and Asp109 of EF-Tu. The crystallographic model is shown with solid lines. Full size image The MD simulations of the ribosome bound EF-Tu complex were generally very stable and it is particularly worth commenting on the fact that several counter ion positions in the neighbourhood of the GTPase catalytic centre appear to be critical for structural integrity, although counter ions were not included in the crystallographic model [8] . One octahedrally coordinated counter ion was modelled here as a K + ion, on the basis of ligand distances in the crystal structures of the free EF-Tu ternary complexes [19] , [20] , where ammonium salt was used in the crystallization medium (K + and NH 4 + have similar radii). This ion is ligated by both Asp50 and Glu55, and appears to be essential for maintaining local structural stability in that region (about 9 Å away from the GTP γ-phosphate). It is further remarkable that the two Mg 2+ ions predicted to be closest (~10Å) to the γ-phosphorous atom (apart from the catalytic Mg 2+ coordinated directly to GTP) correspond to significant positive electron density peaks in the 2F o -F c map calculated from experimental data ( Fig. 2c ). Also these ions have key roles in neutralizing interactions between negatively charged groups, notably RNA backbone phosphates and carboxylate groups of EF-Tu. Note that it is not unusual with flexible sidechains (with high B-factors) being out of density at this resolution as is the case with, for example, Asp21 ( Fig. 2c ), which in the MD simulations is surrounded by several water molecules (not shown). Hence, the importance of a consistent treatment of solvent molecules and counter ions in MD simulations of ribosome complexes must be emphasized as erroneous positions of these are likely to cause both structural and energetic problems. It further appears necessary to compare simulation results to the experimental electron density rather than just to the crystallographic structural model. For example, in most of the independent MD simulations we observed convergence of the Gly83-His84 backbone conformation to that found in the high-resolution structures of the ternary complex [19] , [20] ( Fig. 2b ), which fits equally well into the 3.2 Å density map of the ribosome complex, while the sidechain of His84 remains in the activated state. The limited structural details available in an earlier report [17] do not permit structural comparisons with the MD simulations of GTP hydrolysis by EF-Tu. Free energy calculations With the MD simulations providing stable, reliable structures, it becomes possible to address the energetics of the different process (1)–(4) with a high degree of confidence. The standard reaction-free energies for the proton transfer reactions (1)–(3) in water contain both intrinsic gas-phase and solvation contributions, and are experimentally given by (for example, kcal mol −1 at 25 °C based on p K a of 15.7 and 6.5 for water and histidine, respectively. A similar value of about 12 kcal mol −1 is obtained for proton transfer to GTP in water). The changes in these reaction-free energies upon moving donor and acceptor into the GTPase centre on the ribosome are obtained here by computationally transforming reactants to products, both in water and in the ribosomal environment, using MD/FEP simulations. These relative free energies, , thus directly estimate the change in stability of the hydroxide ion states compared with aqueous solution. Note that the reference reaction in solution for mechanisms (2)–(4) includes a Mg 2+ ion bound to GTP in accordance with experimental data [21] , but not the histidine, while the corresponding reference reaction for (1) does not include GTP. The results from our calculations are summarized in Table 1 , where it can be seen that proton transfer from the bridging water molecule to His84 is greatly disfavoured by over 17 kcal mol −1 , mainly due to the strong repulsion between OH − and the doubly negatively charged γ-phosphate group of GTP. Hence, it would seem impossible for His84 to act as a general base in the hydrolysis reaction. In contrast, proton transfer from the water molecule to the γ-phosphate is clearly facilitated in the ribosomal environment with His84 protonated, compared with aqueous solution, and the ROPO 3 H − +OH − state is stabilized by about 4 kcal mol −1 partly due to the ionic interaction with His84. If the histidine is neutral, on the other hand, there is a considerable destabilization (+16 kcal mol −1 ) of proton transfer to the γ-phosphate ( Table 1 ) and no favourable interaction between the hydroxide and His84 exists as the histidine is deprotonated at the δ1 nitrogen. With a protonated His84 the GTPase active site becomes perfectly arranged for favourable interaction with a hydroxide ion as can be seen in Fig. 3a . The peptide backbone of the PGH motif, which ends with His84, provides an ‘oxyanion hole’ like structure for stabilizing negative charge together with the histidine sidechain, when it is in the active conformation. One can note that this PGH motif is also strictly conserved in all the translational GTPases [22] . Table 1 Comparison of the calculated reaction energetics (kcal mol −1 ) for different possible protonation states involved in GTP hydrolysis by EF-Tu on the ribosome. 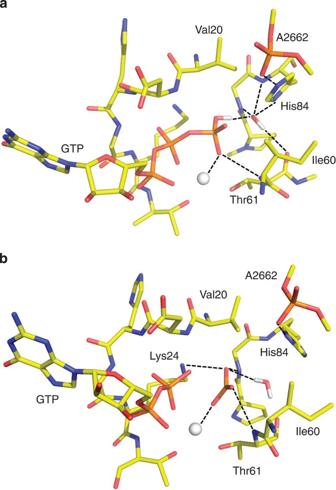Figure 3: Stabilizing interactions in the active site. (a) Representative MD structure of the GTPase centre with a hydroxide ion resulting from proton transfer from water to the γ-phosphate group of GTP. The hydroxide is coordinated by backbone NH groups of the PGH motif, the protonated His84 sidechain, the Thr61 carbonyl group and the now protonated γ-phosphate. (b) MD structure of the transient metaphosphate species in the active site. This is coordinated by Lys23, the backbone NH groups of Thr61 and Gly83, the catalytic water and the GTP bound Mg2+ion (white sphere). Full size table Figure 3: Stabilizing interactions in the active site. ( a ) Representative MD structure of the GTPase centre with a hydroxide ion resulting from proton transfer from water to the γ-phosphate group of GTP. The hydroxide is coordinated by backbone NH groups of the PGH motif, the protonated His84 sidechain, the Thr61 carbonyl group and the now protonated γ-phosphate. ( b ) MD structure of the transient metaphosphate species in the active site. This is coordinated by Lys23, the backbone NH groups of Thr61 and Gly83, the catalytic water and the GTP bound Mg 2+ ion (white sphere). Full size image The stabilization of the resulting protonation state of reaction (2), which would be expected for an associative substrate-assisted mechanism, thus speaks in favour of such a reaction pathway. Interestingly, however, also the limiting case of a dissociative mechanism with a transient metaphosphate species residing between the water nucleophile and the leaving GDP moiety is stabilized by the ribosomal environment by a similar amount (−3.4 kcal mol −1 ). In this case, however, there is no strong interaction between the metaphosphate and the His84 sidechain or the above mentioned oxyanion hole, which now accommodates the neutral water nucleophile ( Fig. 3b ). Instead the (transient) metaphosphate is mainly stabilized by interactions with Lys24, the backbone NH groups of Thr61 and Gly83, as well as the substrate bound Mg 2+ ion. From these simulation results, we can conclude that both the associative and dissociative alternatives for the mechanism of GTP hydrolysis in the EF-Tu complex with the ribosome appear viable, as long as proton transfer to the histidine is not involved. It should also be kept in mind that either neutral water attack on the γ-phosphate dianion or hydroxide ion attack on the monoanion is generally considerably faster than hydroxide attack on the dianion [10] , also suggesting that these mechanistic alternatives are more likely to be operational. As a further check, we also evaluated the energetics of reactions (2) and (4) on the ribosome with His84 in the inactive conformation that it has in the free EF-Tu ternary complex [19] , [20] . That is, while it is clear that reaction (2) and (4) are more favourable than (1), by over 20 kcal mol −1 , the absolute energetics of (2) and (4) may be somewhat difficult to estimate accurately based on comparison to simple reference reactions in water. In contrast, the relative effects associated with transition from the active to non-active state of His84 on the ribosome should be easier to estimate quantitatively as they involve a much smaller perturbation to the system than moving the reactants to aqueous solution. These calculations show ( Table 1 ) that the non-active conformation of His84 causes a destabilization of reaction (2) of about 11 kcal mol −1 compared with the activated structure (hence, the local p K a difference between the water and GTP is reduced by about 8 p K a units upon activation). This value is, in fact, in good agreement with the overall catalytic effect on GTP hydrolysis of EF-Tu on the ribosome [5] . The non-active conformation of His84 also has a detrimental effect of about 4 kcal mol −1 on the dissociative reaction (4), which is smaller than for the substrate-assisted case but still significant. We, furthermore, calculated the p K a difference between His84 in the active and inactive conformations, which yielded an upshift of 2.4±0.5 p K a units for the active form. Assuming that the inactive conformation has an unperturbed p K a this would mean that the activated His84 has a p K a of about 9. This value is thus consistent the observed pH-independence in the 6.5–8.5 pH range for the GTP-γ-S substrate [5] . Structural analysis of protonation states The question of what type of protonation state the crystal structure of the EF-Tu·GDPCP ribosome complex [8] actually corresponds to can also be addressed by structural analysis of MD trajectories. To this end, we first examined ensembles of MD structures from several independent simulations of the key possible protonation states and compared these to the electron density map calculated from the experimental structure factors [8] . This analysis shows that the crystal structure of the EF-Tu·GDPCP ribosome complex most likely corresponds to the resting state with , and not , as can be seen from the MD structures in Fig. 4a . In the former case, the agreement with the crystallographic data is remarkably good ( Fig. 4a ) with the water molecule stably residing between the γ-phosphate group and His84. Just as would be predicted from Fig. 1a , the water donates one H-bond to the phosphate and one to the carbonyl group of Thr61 while receiving an H-bond from the protonated histidine. In the state there is a significant shift of the OH − towards Tyr87 and away from the γ-phosphate due to electrostatic repulsion, reflecting the difficulty of nucleophilic attack of hydroxide ion on the phosphate dianion [10] ( Fig. 4b ). It is also worth examining the predicted structures the state, corresponding to the unlikely possibility that His84 is not protonated (despite it being surrounded by several negative charges). In this case, the nucleophilic water molecule still consistently (just as in the state) donates a hydrogen bond to the γ-phosphate ( Fig. 4c ) and not to the Thr61 carbonyl group as predicted from the crystal structure [8] . Hence, the orientation of the water molecule with a neutral His84 appears suboptimal for attack on the phosphate group and reflects its propensity for proton transfer to it. This is the structure depicted as the active one in Adamczyk and Warshel [17] . It can be noted here that crystallographic position of the water molecule bridging between His84 and GDPCP was obtained from an unbiased F o -F c electron density omit map containing these three groups [8] , while the regular 2F o -F c map apparently has no density for the water position. While the predicted structures of the putative hydroxide ion state were seen to deviate from the experimental data, the MD simulations, in contrast, show that proton transfer to the γ-phosphate according to reaction (2) results in a stable position of the hydroxide that also agrees well with the crystal structure ( Fig. 4d ). This reflects the stable binding position of the hydroxide ion in the above-mentioned oxyanion hole like structure formed by the PGH motif with a protonated His84. In this case, the hydroxide ion also consistently retains its hydrogen bond to the carbonyl group of Thr61 ( Fig. 3a ). 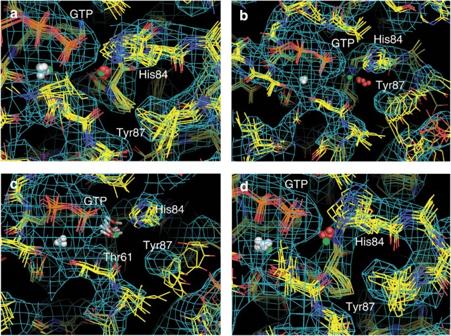Figure 4: Comparison of MD structures with experiment for different protonation states. View of final MD structures of the GTPase centre from (6–10) independent simulations of the states with (a) deprotonated GTP, a neutral water molecule and protonated His84, (b) deprotonated GTP, a hydroxide ion and protonated His84, (c) deprotonated GTP, a neutral water and neutral His84, and (d) protonated GTP, a hydroxide ion and protonated His84. MD positions of the hydrolytic water molecule and GTP bound Mg2+ion are shown as red and white spheres, respectively, while the corresponding crystallographic positions are indicated by green spheres. Incthe catalytic water molecule is shown in stick representation to illustrate its consistent orientation in the simulations. Experimental electron density mesh (2Fo-Fc) calculated from the PDB structure factors (2XQD, 2XQE) (8) is shown in cyan. Figure 4: Comparison of MD structures with experiment for different protonation states. View of final MD structures of the GTPase centre from (6–10) independent simulations of the states with ( a ) deprotonated GTP, a neutral water molecule and protonated His84, ( b ) deprotonated GTP, a hydroxide ion and protonated His84, ( c ) deprotonated GTP, a neutral water and neutral His84, and ( d ) protonated GTP, a hydroxide ion and protonated His84. MD positions of the hydrolytic water molecule and GTP bound Mg 2+ ion are shown as red and white spheres, respectively, while the corresponding crystallographic positions are indicated by green spheres. In c the catalytic water molecule is shown in stick representation to illustrate its consistent orientation in the simulations. Experimental electron density mesh (2F o -F c ) calculated from the PDB structure factors (2XQD, 2XQE) ( [8] ) is shown in cyan. Full size image We further attempted to model the activation process, that is, the conformational change of His84, by running unbiased MD simulations of the ribosome complex starting from the inactive conformation of His84 observed in the free EF-Tu ternary complex [19] , [20] , but retaining the overall conformation of EF-Tu on ribosome [8] . Remarkably, within five independent MD trajectories, totalling 30 ns of simulation time, three activation events were observed. These show that the His84 sidechain, spontaneously, first rotates and then slides into the slot lined by Val20 and Ile60 to make contact with the SRL and approach the GTP γ-phosphate ( Fig. 5 ). Hence, we can conclude that while the overall activation of EF-Tu on the ribosome may be a slower process [5] due to repositioning of its domains relative to each other, the final step of activation where His84 enters into the GTPase centre appears to be rather fast. With a neutral His84, on the other hand, no such activation events are observed, suggesting that protonation of the histidine indeed facilitates its movement into the active conformation. 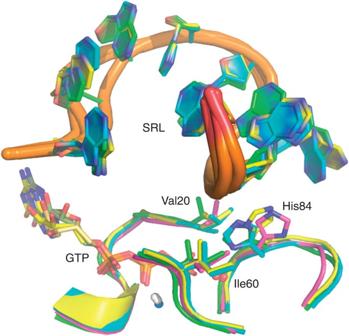Figure 5: Activation of His84. The spontaneous activation of His84 observed during MD simulations is represented by four structures corresponding to the initial unactivated state (magenta carbons),19an intermediate His84 rotated state (yellow carbons) and the final activated state (cyan carbons) superimposed on the corresponding crystallographic structure (green carbons). The SRL is shown as a cartoon with orange backbone in all cases and the hydrophobic gate composed of Val20 and Ile60 is indicated. The overall movement of the His84 Cε1carbon atom is about 5 Å. Figure 5: Activation of His84. The spontaneous activation of His84 observed during MD simulations is represented by four structures corresponding to the initial unactivated state (magenta carbons), [19] an intermediate His84 rotated state (yellow carbons) and the final activated state (cyan carbons) superimposed on the corresponding crystallographic structure (green carbons). The SRL is shown as a cartoon with orange backbone in all cases and the hydrophobic gate composed of Val20 and Ile60 is indicated. The overall movement of the His84 C ε1 carbon atom is about 5 Å. Full size image Effects of mutations Finally, we examined the effect of three EF-Tu mutations on the energetics of proton transfer to the γ-phosphate group (reactions (2) and (3) above), namely His84Ala, His84Arg and His84Gln. The first of these removes the histidine sidechain, thereby allowing more solvent to enter the reaction centre ( Fig. 6 ). Accordingly, the calculated kcal mol −1 predicts a destabilization of the reaction similar to that of the inactive His84 conformation and in agreement with the overall reduction of the GTP hydrolysis rate reported by Rodnina and coworkers [5] . It is also noteworthy that the effect of removing the His84 sidechain is predicted to be less severe than retaining it with the neutral protonation state ( Table 1 ). The second mutation (His84Arg) was chosen as it replaces histidine by another charged sidechain. However, for longer and more flexible sidechains, such as arginine, modelling its conformation in the ribosome complex is not trivial and several conformers may have to be considered. Here, we find two possible conformations of Arg84 that can fit into the active site, corresponding to the g − g + tt and g − tg − g − sidechain rotamers ( Fig. 6 ). These give values of and kcal mol −1 , respectively. Hence, while the first conformation predicts a destabilization of the reaction by 5.3 kcal mol −1 compared with the wild type, the second arginine conformation yields the same result as for His84. The more favourable energetics of the latter appears to be associated with its N ε H group being oriented towards the charge stabilizing (‘PGH’) cavity ( Fig. 6 ) and this g − tg − g − conformation is among the statistically most prevalent rotamers for arginine [23] . It is further interesting that both of the arginine conformers are predicted to yield more favourable energetics than either the His84Ala mutant or inactive His84 conformation, which appears to corroborate the stabilizing effect of a positive charge near the reaction site. Hence, provided that the arginine sidechain actually enters the active site it seems possible that this mutant would retain measurable GTP hydrolysis activity. 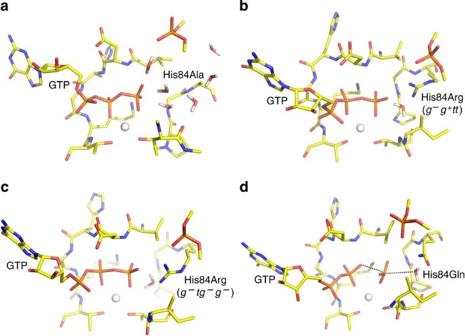Figure 6: Structures of EF-Tu mutants. Predicted structures from MD simulations of the (a) His84Ala, (b,c) His84Arg and (d) His84Gln mutations. For arginine, two conformations are potentially possible in the reaction centre of the ribosomal complex and these correspond to the (b)g−g+ttand (c)g−tg−g−arginine sidechain rotamers. The glutamine mutation (d) is depicted in the state with a transient metaphosphate (partial bonds indicated with dotted lines). The view in all cases is essentially the same as inFig. 3with the same residues depicted. Figure 6: Structures of EF-Tu mutants. Predicted structures from MD simulations of the ( a ) His84Ala, ( b , c ) His84Arg and ( d ) His84Gln mutations. For arginine, two conformations are potentially possible in the reaction centre of the ribosomal complex and these correspond to the ( b ) g − g + tt and ( c ) g − tg − g − arginine sidechain rotamers. The glutamine mutation ( d ) is depicted in the state with a transient metaphosphate (partial bonds indicated with dotted lines). The view in all cases is essentially the same as in Fig. 3 with the same residues depicted. Full size image The GTPase activity of the third EF-Tu mutant, His84Gln, has also been measured experimentally, for T. thermophilus ribosomes at 37 °C, and the results indicate its activity is reduced by a factor of 12 compared with the wild type [6] . The overall stimulation of wild-type GTPase activity upon ribosome binding in that assay was, however, only 50-fold, which might be due to a suboptimal temperature and the use of a yeast Phe-tRNA Phe ( [6] ). The remaining activity for His84Gln is hence not much above the background measured for EF-Tu without tRNA and with unprogrammed 70S ribosomes, which may render the estimate somewhat uncertain. Interestingly, the simulations of proton transfer to the γ-phosphate group with His84Gln yield kcal mol −1 , which is about as unfavourable as for His84Ala, indicating that this variant would be completely inactive. However, it turns out that the glutamine sidechain can instead stabilize the alternative (transient) metaphosphate configuration ( Fig. 6 ) and the calculated value for reaction (4) with the His84Gln mutant is kcal mol −1 . This is about 2 kcal mol −1 more favourable than the reference reaction in water and 1.4 kcal mol −1 less favourable than the effect of the wild type with protonated His84 on the same reaction. This would thus suggest that the observed activity of the His84Gln variant might reflect a shift of the GTP hydrolysis mechanism towards a more dissociative path. The computer simulations based on the existing crystal structure of the EF-Tu·GDPCP ribosome complex [8] carried out here show that the mechanism where His84 acts as general base is highly unlikely due to a large destabilization of the resulting ion pair with a hydroxide close to the γ-phosphate. A concerted GTP hydrolysis mechanism, with nucleophilic attack and proton abstraction by His84 occuring simultaneously, also seems highly improbable for two reasons. First, the catalytic water molecule is seen in the MD simulations to be suboptimally oriented for nucleophilic attack on the phosphate when His84 is in its neutral form and its orientation does not correspond to that predicted from the crystal structure [8] . Second, as the calculated destabilization of the reaction along the stepwise pathway is so large it is very difficult to see how this would be remedied by a concerted mechanism [12] , [13] . Instead, the calculations show that the most favourable proton transfer event is from the water molecule to the γ-phosphate in the presence of a positively charged histidine, in line with the suggestion by Liljas et al . [9] . This process corresponds to the initial step in the limiting case of a fully stepwise associative GTP hydrolysis mechanism, but the energetics of a more concerted associative pathway is still expected to reflect the energetics of the stepwise path as the overall free energy surface often has been found to be rather flat [12] , [13] . Furthermore, the large predicted effect of having His84 in the active as opposed to non-active conformation, which agrees well with the overall catalytic effect of activated EF-Tu measured experimentally [5] , clearly speaks in favour of this type of GTP hydrolysis mechanism that also is congruent with proposals for other GTPases [14] , [15] , [16] . However, the free energy calculations also show that ribosome complex can stabilize a transient metaphosphate species such as would be expected for a fully dissociative hydrolysis mechanism. The effect of His84 is, however, predicted to be considerably smaller in this case, which may cast some doubt on the feasibility of such a reaction path. The concerted mechanism considered in Adamczyk and Warshel [17] appears to lie in between the fully associative and dissociative paths. With regard to the detailed GTP hydrolysis mechanism, it is important to emphasize that our main objective here was to determine whether His84 can act as general base or not , rather than to elucidate the overall reaction pathway. While this can, in principle, be done by QM/MM or empirical valence bond methods, accurate transition state modelling for the rather complex GTP hydrolysis reaction in the highly charged environment of the ribosome is inherently associated with some uncertainties. In this respect, the aforementioned problem of attaining accurate solvent and ion positions is particularly pertinent as, especially, inaccurate counter ion positions can completely obscure the results. We thus consider it more reliable to first evaluate the relative energetics of the well-defined states of the elementary processes (1)–(4) above, as this can be done with straightforward MD/FEP simulations using standard force field parameters. The results of the present calculations also confirm the usefulness of this strategy and clearly show that His84 cannot act as a general base in the reaction. A requirement is, of course, that the MD simulations are carefully gauged against experimental data and in our case we find that comparisons to the actual electron density is necessary when dealing with structures of low resolution (~3Å). Our MD/FEP simulations further reveal that His84 provides an important electrostatic and hydrogen bonding contribution to the catalytic effect in the activated EF-Tu·GTP ribosome complex. Remarkably, direct MD simulations also show how interaction with the SRL spontaneously drives His84 into the activated conformation for GTP hydrolysis. Further, the PGH motif that ends with His84 provides an oxyanion hole like structure, together with the Thr61 backbone NH group and His84 sidechain, which is perfectly adapted for accommodating negative charge ( Fig. 3 ). This cavity will stabilize not only a hydroxide ion but also the leaving phosphate group product, consistent with the experimental finding that P i release is slower than the preceding GTP hydrolysis step ( k Pi =23 s −1 versus k GTP >500 s −1 ) ( [24] ). In fact, any late product-like transition state, resulting from either associative or dissociative mechanisms, is likely to be stabilized by the structural motif (a stable phosphate ion trapped by the PGH motif has also been observed in a crystal structure of aIF2) ( [25] ). This is in contrast to the prediction in Adamczyk and Warshel [17] , whereby the active conformation of the EF-Tu ribosome complex is predicted to destabilize the bound product state (GDP+P i ) by over 20 kcal mol −1 compared with the non-activated state. The predicted endothermicity of the chemical GTP hydrolysis step (7 kcal mol −1 ) ( [17] ), together with the experimental rate of P i release (23 s −1 ) would lead to a composite rate for elongation (after codon recognition) of about 10 −4 s −1 , which is considerably slower than experimentally measured rates [5] . We note that the PGH motif is universally conserved and present in both EF-Tu, EF-G, IF2 and RF3, as well as archeal and eukaryotic translational GTPases [22] . Further, the so-called hydrophobic gate consisting of Val20 and Ile60 defines the boundary of the cavity together with Tyr87 ( Figs 3 , 4 ) and these hydrophobic sidechains prevent excessive solvent molecules from approaching the reaction centre. Also these three residues are highly conserved in all translation GTPases [22] . The above results are somewhat contradictory to the conclusion of Adamczyk and Warshel [17] , that His84 contributes an allosteric effect and that electrostatic stabilization originates from a number of other residues in the vicinity of the GTPase centre. If the histidine is positively charged it would seem likely that it has differential interactions with the reactant and transition states as it is only ~4.5 Å away from the γ-phosphate in the activated state, but it was predicted to only have a negligible direct energetic effect [17] . Furthermore, all the residues depicted in Adamczyk and Warshel [17] as having large and significantly different catalytic contributions in the active and non-active states appear to be in essentially identical positions in the high resolution structures of free EF-Tu ternary complexes [19] , [20] and in the ribosome complex [8] . Although Tyr47 and Cys82 were among the proposed important residues in Adamczyk and Warshel [17] , neither are conserved in the family of translational GTPases [22] . Our results rather suggest that it is the universally conserved PGH motif that is the key catalytic factor in EF-Tu. This motif appears ideally suited for stabilizing negative charge upon movement of the protonated His84 into the active site and the role of the motif is likely to be the same in all other translational GTPases. MD simulations Free energies were calculated from MD simulations using the single topology FEP technique, where the different states involved in reactions (1)–(4) were transformed into each other in the ribosome bound complex, as well as in aqueous solution. Initial coordinates were taken from the crystal structure by Voorhees et al . [8] of the ribosome bound EF-Tu ternary complex (PDB codes: 2XQD, 2XQE). All MD simulations were performed essentially as reported earlier [18] , [26] with the MD package Q [27] utilizing the OPLS-AA force field [28] (Macromodel 9.1, Schrödinger LCC, New York). Spherical simulations systems (40 Å in diameter) centered on the γ phosphorous atom of GTP were used and water molecules close to the sphere boundary were subjected to radial and polarization restraints according to the SCAAS model [27] , [29] . With the exception of interior solvent molecules taken from high resolution structures of the free EF-Tu ternary complex [19] , [20] (see Results ), water molecules were added to the simulation sphere using the standard algorithm of the Q programme, in order to obtain the correct density of the system. Mg 2+ counter-ions placed at electrostatic potential minima were added to the system, and charged groups closer than 5 Å from the simulation boundary were neutralized as described earlier [26] to prevent insufficiently screened charges to exert unphysical influence on the system. RNA backbone phosphate charges in this region were also neutralized by counter ion smearing. The MD simulations were carried out with a time step of 1 fs, in combination with the SHAKE [30] procedure for solvent bonds and angles. A 10 Å cutoff for direct non-bonded interactions was employed, with electrostatic interactions beyond the 10 Å cutoff treated by the local reaction field multipole expansion method [31] . No cutoff was applied to non-bonded interactions involving the central part of the system that changes during the FEP transformations (that is, the triphosphate moiety of GTP, the hydrolytic water molecule and the sidechain of His84). The equilibration phase consisted of stepwise heating from 1 K to 300 K while gradually releasing restraints on heavy solute atoms, followed by 800 ps of unrestrained equilibration at 300 K. Each system was then subjected to 1.1 ns of production phase MD for free energy calculations comprising 21 intermediate FEP states. Six to ten replicate simulations were performed for each system with randomized initial velocities reassigned during equilibration according to the Maxwell distribution. The replicates were run both in the forward and backwards transformation directions. Both structural and energetic convergence was found to be quite satisfactory and no systematic hysteresis effects were found. Error bars in Table 1 are given as s.e.m. for the replicate simulations. Free energy calculations The FEP calculations of reactions (1)–(4) involve creating/annihilating protons, redistributing charge and changing relevant bonded parameters, all given by the OPLS-AA force field. Non-bonded van der Waals parameters for the hydroxide ion, with charges −1.2 (O) and +0.2 (H), were taken from Åqvist’s early work [32] that yielded reliable hydration properties in terms of radial distribution function and solvation energy ( kcal mol −1 ). Charges for the transient metaphosphate species in reaction (4) were +1.1 (P) and −0.7 (O), with standard OPLS-AA phosphate van der Waals parameters. Axial oxygen ligands to the metaphosphate were restrained to a 2.8 Å distance from the phosphorous atom. The solution reference reaction for (1) only includes a histidine residue and a water molecule, while the solution reference reactions for (2)–(4) encompass GTP 4− , Mg 2+ and a water molecule. Proton transfer to either of the two γ-phosphate oxygens not ligated to the Mg 2+ ion was further found to be energetically equivalent. These reference reactions in solution were run using the same protocol as above. For reaction (1) weak harmonic restraints to the crystallographic positions with a force constant of 1.0 kcal mol −1 A −2 ) were applied to the water oxygen and ND1 atom of the histidine, both in the ribosome complex and in water. Corresponding restraints were applied to the γ phosphorous and water molecule in reactions (2) and (3), as well as for the solution reference reaction. Finally, each of the replicate simulations for the ribosome systems were then further prolonged without any restraints applied in order to gauge the stability of the hydrolytic water/hydroxide positions ( Fig. 4 ). Spontaneous activation of the His84 sidechain was monitored by running several independent MD simulations starting from the structure of ribosome bound EF-Tu ternary complex [8] , but with His84 in the inactive conformation that it has in the free ternary complex [19] . This was done for the protonated and unprotonated forms of His84 with 30–32 ns of MD simulation for each system. The p K a shift between active and inactive conformations was calculated from their respective electrostatic free energy differences between the neutral and protonated forms utilizing the linear response approximation [33] , . Here, denotes the average electrostatic interaction energy difference between protonated and unprotonated forms of His84 and the subscripts denote that MD sampling is carried out for both protonation states. Electron density calculations For structural comparisons with the experimental data an electron density map was calculated using standard procedures. The split PDB coordinate files (2XQD, 2XQE) and the structure factor data were downloaded from the PDB. The coordinate files were hand edited to produce one large coordinate file and a structure factor calculation made using a bulk-solvent correction and isotropic scaling [34] with the Phenix system [35] . These calculations produced R work and R free values of 0.236 and 0.271 for all reflections in the resolution range 48–3.01 Å (compared with values of 0.231 and 0.268 for reflections in the range 50–3.1 Å that were reported in the PDB file header). The σ A -weighted (2m|Fo|—D|Fc|) electron-density maps [36] were calculated within Phenix. How to cite this article: Wallin, G. et al . Energetics of activation of GTP hydrolysis on the ribosome. Nat. Commun. 4:1733 doi: 10.1038/ncomms2741 (2013).